Endocannabinoids modulate cortical development by configuring Slit2/Robo1 signalling Local environmental cues are indispensable for axonal growth and guidance during brain circuit formation. Here, we combine genetic and pharmacological tools, as well as systems neuroanatomy in human fetuses and mouse models, to study the role of endocannabinoid and Slit/Robo signalling in axonal growth. We show that excess 2-arachidonoylglycerol, an endocannabinoid affecting directional axonal growth, triggers corpus callosum enlargement due to the errant CB 1 cannabinoid receptor-containing corticofugal axon spreading. This phenotype mechanistically relies on the premature differentiation and end-feet proliferation of CB 2 R-expressing oligodendrocytes. We further show the dependence of both axonal Robo1 positioning and oligodendroglial Slit2 production on cell-type-specific cannabinoid receptor activation. Accordingly, Robo1 and/or Slit2 manipulation limits endocannabinoid modulation of axon guidance. We conclude that endocannabinoids can configure focal Slit2/Robo1 signalling to modulate directional axonal growth, which may provide a basis for understanding impaired brain wiring associated with metabolic deficits and prenatal drug exposure. Axonal pathfinding decisions rely on short- and long-range intercellular cues determining cytoarchitectural arrangements permissive for directional growth in the developing brain. Guidance cues include a plethora of structurally heterogeneous proteins, released during defined temporal windows and acting within circumscribed spatial domains. Slits, a family of phylogenetically conserved chemorepellent molecules [1] , bind Roundabout (Robo)1/2 receptors [2] , [3] to regulate axonal tract formation during forebrain development [4] , [5] , [6] , [7] , [8] . Slit/Robo1/2 signalling is implicated in midline crossing [9] , [10] , [11] , [12] and the dorsoventral positioning of long-range axons [13] , [14] , thus being indispensable for the basic forebrain wiring diagram and connectivity principles to emerge. Accordingly, Robo1 −/− mice present the dysgenesis of major commissural tracts [5] and axon guidance errors in the corticofugal system [4] . Similarly, Slit2 −/− and Slit1 −/− /Slit2 −/− mice show corticothalamic- and thalamocortical-targeting defects [8] , as well as optic tract abnormalities [12] . In addition, axons coalesce into enlarged fascicles in Robo1 −/− mice [5] . Heparin sulphate proteoglycans and transcription factors, including members of the T-box or the LIM homeodomain families can influence Slit/Robo1/2 signalling [14] . Nevertheless, the molecular identity of signalling networks for the upstream and local control of coordinated Slit/Robo1/2 expression, subcellular positioning and signal competence during corticogenesis remains relatively poorly explored. Signalling lipids have recently emerged as regulators of neuronal development. Endocannabinoids, the natural ligands of cannabinoid receptors, modulate both neuronal [15] and glial [16] differentiation, and are efficacious to facilitate neurite extension and growth cone-steering decisions [17] , [18] , [19] . CB 1 cannabinoid receptors (CB 1 Rs) contribute to regulating the fasciculation and pallidal targeting of corticofugal axons [17] . In contrast, CB 2 cannabinoid receptors (CB 2 Rs) are co-expressed with key enzymes of 2-arachidonoylglycerol (2-AG) metabolism in glia [20] , and promote the differentiation of cultured oligodendrocytes [21] , the cellular source of myelin sheaths in the nervous system [22] . Here, we show that pharmacological enhancement of 2-AG bioavailability during corticogenesis in mouse triggers the CB 2 R-dependent differentiation of oligodendrocytes. Premature oligodendrocyte end-feet proliferation in vivo coincides with CB 1 R-dependent fasciculation errors of corticofugal projections, including altered axon bundle formation in the paramedian domain of the corpus callosum. We hypothesized that endocannabinoids, by simultaneously engaging cell-type-specific cannabinoid receptors, might orchestrate chemorepulsion of cortical axons via a mechanism operating in trans , with oligodendrocytes producing surplus chemorepellents. By implementing a multi-parametric approach, encompassing neuroanatomy in human and mouse fetuses, messenger RNA (mRNA) profiling, biochemistry, in vitro analysis and genetic models, we identify oligodendrocyte-derived Slit2 acting at Robo1 receptors in corticofugal axons downstream from the respective activation of CB 2 Rs and CB 1 Rs upon pharmacological manipulation of 2-AG degradation as the molecular underpinning of endocannabinoid-induced corticofugal axon guidance errors. We find cannabinoid receptor activation to facilitate Slit2 accumulation in oligodendrocyte end feet, and Robo1 accumulation in axonal growth cones. Overall, these data suggest that endocannabinoid signalling can regulate Slit/Robo interactions during the establishment of forebrain axonal tracts. JZL184 increases 2-AG levels in fetal and adult cortices To enhance endogenous 2-AG signalling in gravid mice, we employed the small molecule JZL184 from embryonic day (E)12.5–18.5 to inhibit monoacylglycerol lipase (MGL), the enzyme chiefly responsible for degrading 2-AG in the nervous system [23] . The selective inhibition of MGL by JZL184 was confirmed with activity-based protein profiling of serine hydrolases in the brains of JZL184 and vehicle-treated dams and their E18.5 embryos. Consistent with previous reports [24] , JZL184 displayed a high selectivity for MGL across all detectable brain serine hydrolases ( Fig. 1a ) leading to a significant increase in 2-AG levels in adult and embryonic cortices ( Fig. 1b ). While fatty-acid amide hydrolase (FAAH) [25] , which catabolizes the endocannabinoid anandamide (AEA), was partially inhibited by JZL184 in adult and to a lesser degree, embryonic brain samples, we did not observe a significant increase in AEA levels in fetal or adult cortices ( Fig. 1b ). The levels of 2-linoleoyl glycerol (a congener of 2-AG) and oleoylethanolamide (an analogue of AEA), were both unaffected by JZL184 treatment ( Fig. 1b ). Together, these data confirm that JZL184 selectively targets MGL leading to an accumulation of 2-AG in the brains of gravid adult mice and their offspring. 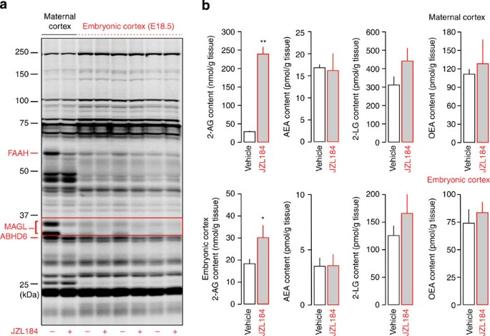Figure 1: JZL184 increases 2-AG levels in maternal and embryonic brains. (a)Ex vivoactivity-based protein profiling of brain-derived serine hydrolases in vehicle and JZL184 (40 mg kg−1)-treated adult and fetal cortices. (b) Select 2-monoacyl glycerol andN-acyl amide levels in maternal and fetal brains correlatively measured after JZL184 treatment. Data were expressed as means±s.e.m.,n=2 per group (mothers),n=6 per group (fetuses); **P<0.01, *P<0.05 (Student’st-test). Figure 1: JZL184 increases 2-AG levels in maternal and embryonic brains. ( a ) Ex vivo activity-based protein profiling of brain-derived serine hydrolases in vehicle and JZL184 (40 mg kg −1 )-treated adult and fetal cortices. ( b ) Select 2-monoacyl glycerol and N -acyl amide levels in maternal and fetal brains correlatively measured after JZL184 treatment. Data were expressed as means±s.e.m., n =2 per group (mothers), n =6 per group (fetuses); ** P <0.01, * P <0.05 (Student’s t -test). Full size image MGL inhibition induces axon fasciculation deficits We studied the morphology of corticofugal axons in developing fetal brains after JZL184 exposure, since these tracts contain the highest levels of CB 1 Rs during embryonic development [18] . JZL184 exposure induced L1 neural cell adhesion molecule (L1-NCAM) + axons to coalesce into enlarged fascicules ( Fig. 2a,b ; Supplementary Table 1 ) irrespective of the rostrocaudal axis of the developing brain ( Supplementary Fig. 1a–c ). The enlarged axon fascicles were found spread in the cortical plate, including intermediate zone territories otherwise devoid of L1-NCAM + processes ( Fig. 2i,j ; Supplementary Fig. 1a ). 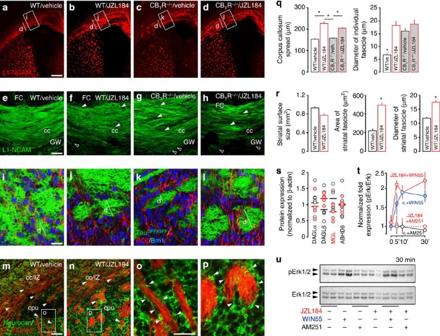Figure 2: JZL184 alters callosal axon fasciculation and pathfinding. (a–d) Corticofugal axonal phenotypes and (e–h) their midline crossing in vehicle- or JZL184-treated mouse embryos at E18.5. (i–l) A taugfp/gfpreporter mouse29was used for the genetic tagging of corticofugal axons. Axon fasciculation errors present in CB1R−/−mice (k), were further increased by JZL184 (surface area occupied by corticofugal axons (l). (m–p) Neurocan was excluded from enlarged axon fascicles in JZL184-exposed brains. (q) Corpus callosum spread in both wild-type and CB1R−/−mice. (r) Striatal surface size, and the cross-sectional surface area and diameter of axon fascicles in JZL184- or vehicle-treated mice. (s) DAGLα, DAGLβ, MGL and ABHD6 protein levels in JZL184-treated (red circles) versus control (open circles) cortices on E18.5. (t,u) Erk1/2 phosphorylation upon acute WIN55,212-2 and/or AM251 stimulation in drug naive and JZL184 pre-treated (4 days) neurons. Data were expressed as means±s.e.m.,n=3/group (q,r).In vitroexperiments were performed in duplicates withn≥2 samples per experiment run in parallel. *P<0.05 (Student’st-test). cc, corpus callosum; cpu, caudate putamen; FC, fiber crossing; GW, glial wedge; IZ, intermediate zone. Scale bar, 300 μm (a–h,m,n), 10 μm (i–l,o,p). Figure 2: JZL184 alters callosal axon fasciculation and pathfinding. ( a – d ) Corticofugal axonal phenotypes and ( e – h ) their midline crossing in vehicle- or JZL184-treated mouse embryos at E18.5. ( i – l ) A tau gfp/gfp reporter mouse [29] was used for the genetic tagging of corticofugal axons. Axon fasciculation errors present in CB 1 R −/− mice ( k ), were further increased by JZL184 (surface area occupied by corticofugal axons ( l ). ( m – p ) Neurocan was excluded from enlarged axon fascicles in JZL184-exposed brains. ( q ) Corpus callosum spread in both wild-type and CB 1 R −/− mice. ( r ) Striatal surface size, and the cross-sectional surface area and diameter of axon fascicles in JZL184- or vehicle-treated mice. ( s ) DAGLα, DAGLβ, MGL and ABHD6 protein levels in JZL184-treated (red circles) versus control (open circles) cortices on E18.5. ( t , u ) Erk1/2 phosphorylation upon acute WIN55,212-2 and/or AM251 stimulation in drug naive and JZL184 pre-treated (4 days) neurons. Data were expressed as means±s.e.m., n =3/group ( q , r ). In vitro experiments were performed in duplicates with n ≥2 samples per experiment run in parallel. * P <0.05 (Student’s t -test). cc, corpus callosum; cpu, caudate putamen; FC, fiber crossing; GW, glial wedge; IZ, intermediate zone. Scale bar, 300 μm ( a – h , m , n ), 10 μm ( i – l , o , p ). Full size image The coalescing of axonal fibres upon JZL184 exposure was altered irrespective of their origin or projection targets. In particular, enlarged fascicles were observed to cross the midline ( Fig. 2e,f ), populated the suprastriatal domain of the corpus callosum ( Fig. 2m,n ; Supplementary Fig. 2a ) or invaded the striatum ( Fig. 2o,p ). Both corticothalamic and thalamocortical axons were affected in the striatum, as revealed by TAG-1 (refs 26 , 27 ) and C-terminal full length of mouse GPR55 (ref. 17 ) immunohistochemistry, respectively ( Supplementary Fig. 2a–e,r ). These findings suggest the multimodal interplay of corticofugal and thalamocortical projections along their reciprocal growth paths during the mechanism termed axonal ‘handshake’ [28] . Next, we examined mice carrying green fluorescent protein (GFP)-tagged cytosolic tau in neurons [29] in the presence or absence of CB 1 Rs (tau gfp/gfp ::CB 1 R) [29] to show that radial glia (RC2 + ) fibres and post-mitotic Brn1 + pyramidal cells [16] arranged perpendicular to corticofugal axons and adopted alternative paths ( Fig. 2i,j ). We then administered JZL184 to CB 1 R −/− fetuses to test the reliance of pharmacologically induced axon guidance errors on CB 1 Rs, selectively localized to the corticofugal system by mid-gestation [18] . In accord with previous reports [18] , [30] , CB 1 R deletion alone induced axon fascicle enlargement ( Fig. 2c,g,k,q ). In CB 1 R −/− animals, JZL184 did not affect the diameter of first-order fascicles (18.78±1.66 μm (JZL184) versus 16.04±1.28 μm (vehicle) (mean±s.e.m. ; n =3 mice per group); Fig. 2d,h,l,q ). CB 1 R −/− mice treated with JZL184 presented significantly increased axon spreading in the intermediate zone/corpus callosum (203.81±8.44 μm (JZL184) versus 157.27±6.28 μm (vehicle), n =3 mice per group, P <0.05 (Student’s t -test); Fig. 2q ). This was associated with altered distribution of radial glia processes and Brn1 + pyramidal cell radially migrating towards the cortical plate—to avoid axon-packed microdomains—in tau gfp/gfp ::CB 1 R −/− reporter mice ( Fig. 2l ). The dynamic control of axonal growth and fasciculation involves the elimination of functionally redundant or mistargeted processes over time. Mature axons become embedded in extracellular matrix, a three-dimensional scaffold of molecularly heterogeneous proteins [31] , to maintain their positions in axon fascicles. Here, we find that neurocan, a chondroitin sulphate proteoglycan whose expression is essential for cell adhesion and slows neurite extension [32] , is excluded from enlarged axonal fascicles upon JZL184 treatment ( Fig. 2m–p ), suggesting altered neurite motility and pathfinding. The JZL184-induced remodelling of the corticofugal system also impacted the coincident patterning of thalamocortical afferents ( Supplementary Fig. 2a–e ), robustly affecting their ‘handshake’ [28] . Nevertheless, the JZL184-induced axonal phenotype was absent in constitutive MGL −/− mice ( Supplementary Fig. 3 ). Chronic 2-AG signalling in MGL −/− mice is characterized by CB 1 R downregulation and desensitization, suggesting compensation for increased CB 1 R signalling events [23] . Inhibition of MGL by JZL84 in our experimental model (E12.5-E18.5) would likely induce excessive CB 1 R signalling, resulting in physiological alterations otherwise compensated for in MGL −/− mice. Thus, we conclude that excess 2-AG availability brought about by the pharmacological disruption of their degradation during defined periods of corticogenesis is sufficient to remodel the corticofugal projection system. Unchanged CB 1 R signal transduction upon JZL184 exposure Repeated JZL184 administration can induce cannabinoid receptor desensitization and functional antagonism [23] . Therefore, we first sampled mRNA ( Supplementary Table 2 ) and protein expression of molecular constituents of the 2-AG signalling cassette ( Fig. 2s ; Supplementary Fig. 4 ). Neither mRNA nor protein levels for sn -1-diacylglycerol lipases α and β (DAGL), synthesizing 2-AG [33] , MGL and ABHD6, involved in 2-AG degradation [34] , [35] , and CB 1 Rs changed significantly in JZL184-exposed fetal cortices ( Supplementary Fig. 4a,b ). We then used extracellular signal-regulated kinase 1/2 (Erk1/2) phosphorylation as a read-out [36] upon acute agonist challenge (WIN55,212-2, 100 nM) of cultured cortical neurons pre-treated with JZL184 for 4 days to address whether JZL184 induced CB 1 R desensitization. JZL184 alone did not induce constitutive Erk1/2 phosphorylation, and AM251, a CB 1 R antagonist, did not modify JZL184 effects. Notably, JZL184 allowed WIN55,212-2-induced rapid Erk1/2 phosphorylation ( Fig. 2t,u ) with comparable temporal dynamics to that in control ( Supplementary Fig. 4c ), which is compatible with earlier data showing that only prolonged (>8 days) agonist stimulation induces CB 1 R desensitization in vitro [36] . These data suggest that supra-physiological 2-AG signals upon JZL184 application during corticogenesis alter axon fasciculation via neuronal CB 1 Rs, while a non-CB 1 R-mediated mechanism might account for the increased axonal spread in the prospective corpus callosum. Oligodendrocyte end feet proliferate among misrouted axons Excessive spreading of corticofugal axons committed to the prospective corpus callosum in JZL184-treated CB 1 R −/− mice led us to hypothesize that a CB 1 R-independent mechanism can alter the pathfinding of corticofugal axons. Therefore, we tested whether premature differentiation of oligodendrocytes, which postnatally produce myelin to ensheath callosal axons [22] and co-express CB 1 Rs and CB 2 Rs [20] , could participate in axonal misrouting. JZL184 facilitated the accumulation of oligodendrocytes that expressed 2′,3′-cyclic-nucleotide 3′-phosphodiesterase (CNPase) [20] , and formed micro-islands interspersed with corticofugal axons in both wild-type and CB 1 R −/− mice ( Fig. 3a–d ). Oligodendrocyte differentiation was reflected by the increased density ( Fig. 3e ) and size ( Fig. 3f ) of their CNPase + end feet targeted towards nearby axons. The JZL184-induced morphogenesis of oligodendrocytes was CB 1 R independent since it also occurred in CB 1 R −/− mice (density: 37. 7±3.1 (JZL184) versus 14.7±2.7 (vehicle) end feet/1,000 μm 2 , P <0.05; Fig. 3e ). By western blotting, we quantitatively confirmed that JZL184 significantly elevated CNPase and myelin basic protein levels in the fetal cerebrum ( Fig. 3g,h ). These results outline a multicomponent mechanism with 2-AG simultaneously activating CB 1 Rs in axons, and CB 2 Rs in oligodendrocytes in JZL184-exposed fetuses. Nevertheless, a causal relationship between altered axonal navigation and glial proliferation remains unknown. Here, we reasoned that endocannabinoid-induced glial differentiation might instruct the production of a chemorepellent for the focal remodelling of the corticofugal tract ( Fig. 3i ). 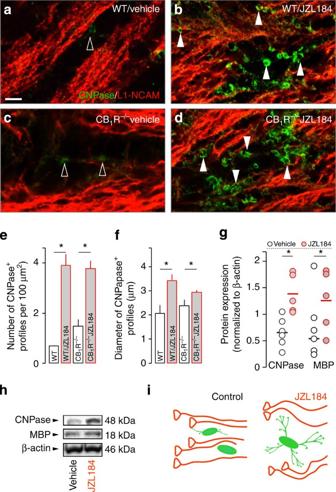Figure 3: JZL184 induces oligodendrocyte differentiation. CNPase+oligodendroyctes in the prospective corpus callosum were infrequently detected in wild-type (a) and CB1R−/−(c) embryos (E18.5; open arrowheads). (b,d) JZL184-induced oligodendrocyte differentiation, which progressed in CB1R−/−mice (solid arrowheads pinpoint end feet). (e,f) Quantitative data on oligodendrocyte morphology. (g,h) CNPase and myelin basic protein (MBP) levels in the cortices of JZL184-treated mouse embryos. (i) Schema of JZL184-induced remodelling of axonal pathfinding upon premature oligodendrocyte differentiation. Data were expressed as means±s.e.m.,n=5/6 (JZL184/vehicle), *P<0.05 (Student’st-test). Scale bar, 4 μm (a). Figure 3: JZL184 induces oligodendrocyte differentiation. CNPase + oligodendroyctes in the prospective corpus callosum were infrequently detected in wild-type ( a ) and CB 1 R −/− ( c ) embryos (E18.5; open arrowheads). ( b , d ) JZL184-induced oligodendrocyte differentiation, which progressed in CB 1 R −/− mice (solid arrowheads pinpoint end feet). ( e , f ) Quantitative data on oligodendrocyte morphology. ( g , h ) CNPase and myelin basic protein (MBP) levels in the cortices of JZL184-treated mouse embryos. ( i ) Schema of JZL184-induced remodelling of axonal pathfinding upon premature oligodendrocyte differentiation. Data were expressed as means±s.e.m., n =5/6 (JZL184/vehicle), * P <0.05 (Student’s t -test). Scale bar, 4 μm ( a ). Full size image CB 1 Rs coexist with Robo1/2 receptors in corticofugal axons Neurons and glia interact to form chemical conduits for axonal growth during brain development [14] . Slit/Robo interplay is fundamental for the development of major axonal tracts, including corticofugal projections [4] , [5] , with midline glia being a primary source of chemorepellent Slit1/2 (ref. 37) [37] . However, the upstream regulation of Slit/Robo signalling in axon guidance is not entirely understood. We hypothesized that endocannabinoid-induced oligodendroglia positioning and differentiation in conjunction with 2-AG’s cell-type-specific action via CB 1 Rs and CB 2 Rs could orchestrate in trans Slit/Robo signalling. Therefore, we first examined whether CB 1 Rs and Robo1 receptors coexist in long-range axons. By using serial sections from human fetuses at gestational weeks 20–23 ( Supplementary Table 3 ), we find the expression patterns of CB 1 Rs and Robo1 receptors to overlap in forebrain axonal tracts, particularly axons coursing in the internal capsule ( Fig. 4a–d ). Multiple immunofluorescence labelling substantiated that CB 1 Rs and Robo1 receptors indeed co-distributed along the same axons in humans ( Fig. 4e–g ). Likewise, corticofugal axons in the E18.5 fetal mouse brain contained both receptors ( Fig. 4h–m ). In addition, CB 1 R + cortical axons in the corpus callosum harboured Robo2 receptors ( Fig. 4n–p ). 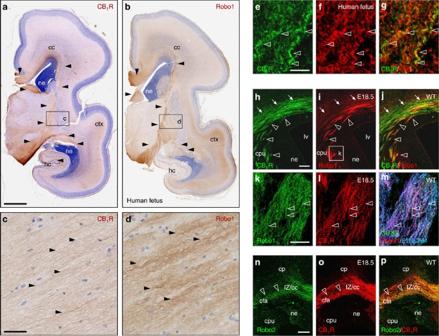Figure 4: CB1Rs co-localize with Robo1 receptors in human and mouse corticofugal axons. (a,b) The regional distribution of CB1R and Robo1 receptor immunoreactivities in human fetal serial sections (closed arrowheads). (c,d) CB1R and Robo1 receptor immunoreactivities in corticofugal fibres in the internal capsule at high magnification. (e–g) Co-localization of CB1R and Robo1 receptors in human fetal tissues (internal capsule) by high-resolution laser-scanning microscopy (open arrowheads). Robo1 (h–m), as well as Robo2 (n–p), were co-expressed with CB1Rs in mouse callosal axons (arrowheads). cc, corpus callosum; cfa, corticofugal axons; cp, cortical plate; cpu, caudate putamen; hc, hippocampus; IZ, intermediate zone; ne, neuroepithelium. Scale bar, 3 mm (a), 200 μm (h,n), 40 μm (c), 7 μm (k). Figure 4: CB 1 Rs co-localize with Robo1 receptors in human and mouse corticofugal axons. ( a , b ) The regional distribution of CB 1 R and Robo1 receptor immunoreactivities in human fetal serial sections (closed arrowheads). ( c , d ) CB 1 R and Robo1 receptor immunoreactivities in corticofugal fibres in the internal capsule at high magnification. ( e – g ) Co-localization of CB 1 R and Robo1 receptors in human fetal tissues (internal capsule) by high-resolution laser-scanning microscopy (open arrowheads). Robo1 ( h – m ), as well as Robo2 ( n – p ), were co-expressed with CB 1 Rs in mouse callosal axons (arrowheads). cc, corpus callosum; cfa, corticofugal axons; cp, cortical plate; cpu, caudate putamen; hc, hippocampus; IZ, intermediate zone; ne, neuroepithelium. Scale bar, 3 mm ( a ), 200 μm ( h , n ), 40 μm ( c ), 7 μm ( k ). Full size image Robo1 accumulates in JZL184-exposed neuronal growth cones Axonal growth is a dynamic process, with growth cones continuously sampling the local microenvironment and responding to chemotactic cues by initiating turning decisions [38] . Robo1/2 localization to growth cones underpins Slit/Robo signalling during axonal pathfinding [13] , [39] . On the basis of our pharmacological data ( Supplementary Fig. 4d ), we hypothesized that modifications to axonal growth trajectories might be mediated by the CB 1 R-dependent repartitioning of Robo1 receptors in axonal growth cones. Therefore, we confirmed the co-localization of CB 1 Rs and Robo1 receptors in vitro ( Fig. 5a ), and validated Robo1/2 mRNA and protein expression by PCR ( Fig. 5b ) and western blotting ( Fig. 5c ). Upon JZL184 treatment of cultured cortical neurons, Robo1 receptors accumulated in growth cones, specified as the fluorescence ratio between the growth cone and adjoining neurite shaft ( Fig. 5d ). This response was O-2050 sensitive [30] , confirming CB 1 R involvement. In contrast, Robo2 receptor distribution remained unchanged ( Fig. 5e ). We also found a decreased co-localization coefficient for Robo1 and CB 1 R, reinforcing increased Robo1 receptor import if CB 1 R levels remained stationary and partition separately from Robo1 ( Fig. 5f ; Supplementary Fig. 5a ). Next, we purified growth cone particles (GCPs) [19] from fetal mouse cortices treated en-block with JZL184 (100 nM) up to 80 min to highlight the in vivo relevance of our findings. Robo1 receptor accumulated in JZL184-exposed GCPs ( Fig. 5g ), lending further support to the concept that superfluous 2-AG signalling can redistribute Robo1 receptors in a CB 1 R-dependent fashion. Furthermore, we suggest that axonal transport contributes to Robo1 accumulation in growth cones, since we detected a JZL184-induced increase in Robo1 receptor immunofluorescence in the distal (presumed motile) [30] part of the neurite adjacent to the growth cone ( Fig. 5h ). 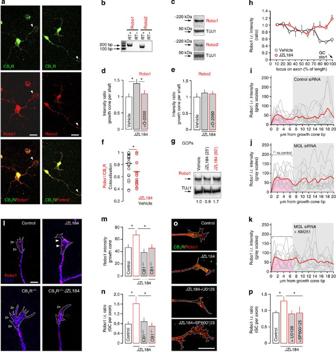Figure 5: CB1R stimulation regulates subcellular Robo1 positioning. (a) Robo1 and Robo2 immunoreactivity in the somata and neurites (including growth cone; arrowheads) of CB1R+cortical neuronsin vitro. (b,c) Cultured cortical neurons expressed both Robo1/Robo2 mRNA and protein. (d) Robo1 and Robo2 (e), fluorescence intensity in growth cones treated with JZL184 or O-2050, a CB1R antagonist. (f) Co-localization coefficient of Robo1 and CB1R in growth cones upon JZL184 exposure. (g) JZL184 induced Robo1 accumulation in growth conesex vivoin isolated growth cone particles (GCPs). (h) Robo1 immunoreactivity adjacent to the growth cone in JZL184-treated neurons. (i–k) Robo1 immunoreactivity in growth cones upon siRNA-mediated MGL silencing in cultured primary neurons. (l–n) Effect of the genetic ablation of CB1Rs in cortical neurons on Robo1 receptor expression in growth cones after JZL184 or vehicle administration. (o,p) The effect of Erk1/2 (U0126) and JNK1 (SP600125) inhibition on Robo1 distribution. Data were expressed as means±s.e.m., from triplicate experiments (sample size: 8–25 neurons per group in morphometric analysis), *P<0.05 (Student’st-test). Scale bar, 10 μm (a), 5 μm (l,o). Figure 5: CB 1 R stimulation regulates subcellular Robo1 positioning. ( a ) Robo1 and Robo2 immunoreactivity in the somata and neurites (including growth cone; arrowheads) of CB 1 R + cortical neurons in vitro . ( b , c ) Cultured cortical neurons expressed both Robo1/Robo2 mRNA and protein. ( d ) Robo1 and Robo2 ( e ), fluorescence intensity in growth cones treated with JZL184 or O-2050, a CB 1 R antagonist. ( f ) Co-localization coefficient of Robo1 and CB 1 R in growth cones upon JZL184 exposure. ( g ) JZL184 induced Robo1 accumulation in growth cones ex vivo in isolated growth cone particles (GCPs). ( h ) Robo1 immunoreactivity adjacent to the growth cone in JZL184-treated neurons. ( i – k ) Robo1 immunoreactivity in growth cones upon siRNA-mediated MGL silencing in cultured primary neurons. ( l – n ) Effect of the genetic ablation of CB 1 Rs in cortical neurons on Robo1 receptor expression in growth cones after JZL184 or vehicle administration. ( o , p ) The effect of Erk1/2 (U0126) and JNK1 (SP600125) inhibition on Robo1 distribution. Data were expressed as means±s.e.m., from triplicate experiments (sample size: 8–25 neurons per group in morphometric analysis), * P <0.05 (Student’s t -test). Scale bar, 10 μm ( a ), 5 μm ( l , o ). Full size image JZL184-induced alterations in Robo1, but not Robo2 protein expression, were rescued by OMDM188, an inhibitor of DAGLs producing 2-AG [40] , implicating 2-AG dependence of Robo1 signalling ( Supplementary Fig. 4d,e ). Therefore, we focused on the endocannabinoid dependence of Slit2/Robo1 interactions. To confirm the reliance of our proposed mechanism on MGL activity, we transfected primary cortical neurons with MGL short interfering RNA (siRNA) and assessed Robo1 receptor intensity in the growth cone. Transient MGL knockdown recapitulated the accumulation of Robo1 immunoreactivity within the growth cone ( Fig. 5i,j ; Supplementary Fig. 5d,e ), which was CB 1 R dependent given its sensitivity to AM251, a CB 1 R inverse agonist ( Fig. 5k ). In addition, the lack of Robo1 receptor responsiveness in the growth cones of primary cortical cultures from CB 1 R −/− mice reinforced the critical involvement of CB 1 Rs in this regulatory process ( Fig. 5i–n ). CB 1 R activation in developing neurons triggers molecularly diverse second-messenger cascades [41] . Here, we found that JZL184-induced Robo1 receptor accumulation in growth cones was occluded by the administration of both U0126 and SP600125, MEK1/2 and c-Jun N-terminal kinases (JNK) inhibitors, respectively ( Fig. 5o,p ). If a CB 1 R-mediated increase of Robo1 signalling is of pathophysiological significance, then Robo/Slit mRNA levels might be expected to coordinately change in the cortices of human fetal subjects exposed in utero to cannabis, relative to controls. By using the NanoString technology ( Supplementary Table 4 ), we found that Robo1 receptor mRNA expression tended to be significantly higher in cannabis-exposed subjects ( F 1,26 =4.156; P =0.056; Supplementary Fig. 1d ). This change was driven by a significant impact of developmental growth measures. Similarly for Slit1 mRNA, there was a significant confound of development resulting in only a trend effect ( P =0.093) for the contribution of cannabis exposure. Interestingly, there was a significant correlation ( r =0.576; P =0.002) between the expression of Robo1 and Slit1 mRNAs in the human fetal cortex, suggesting a functional interaction irrespective of cannabis predisposition. JZL184 promotes Slit2 production in oligodendrocytes Genetic deletion of Slit1 and/or Slit2 induces midline crossing errors [8] , [12] . Therefore, we hypothesized that oligodendrocytes could produce excess Slits in a CB 2 R-dependent fashion to impact corticofugal axon fasciculation. Owing to methodological constraints to histochemically detect Slit1, we adopted a candidate approach and focused on Slit2 throughout our proof-of-concept experiments. We first prepared oligodendrocyte cultures, which only sporadically contained astroglia ( Fig. 6a ) to demonstrate that CNPase + oligodendrocytes are a likely source of Slit2 in vitro . We extended these data by comparing glial fibrillary acidic protein (GFAP) + astroglia and oligodendroglia cultures ( Fig. 6b ), and showing that oligodendroglia selectively contain detectable Slit2 mRNA transcripts and Slit2-like protein ( Fig. 6c ; Supplementary Figs 5b and 6 ). Slit2-like immunoreactivity was seen only in oligodendrocytes (but not astroglia or neurons; Fig. 6a ) in vitro and mainly localized to their soma ( Fig. 6d ) and membranes of their processes ( Fig. 6e,f ). We confirmed our Slit2 detection in oligodendrocytes by demonstrating significantly diminished Slit2-like content in oligodendroglia from Slit2 −/− mice ( Supplementary Fig. 6a–e ). In addition, we validated our staining protocols by co-labelling for an antibody revealing a phylogenetically conserved sequence from the Drosophila Slit ortholog ( Fig. 6c ). These data identify oligodendrocytes as a candidate source of Slit2. 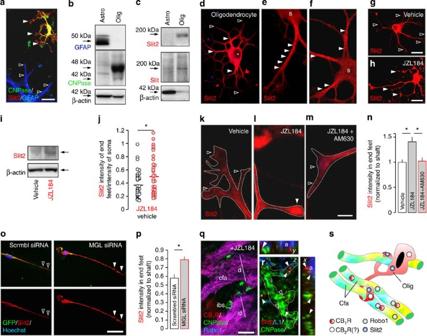Figure 6: JZL184 alters Slit2 expression and localization in oligodendrocytes. (a) Oligodendrocytes (solid arrowheads), but not astrocytes, (open arrowheads) contained Slit2. (b) GFAP and CNPase were used to validate the purity of isolated astrocytes and oligodendrocytes, respectively. (c) Oligodendrocytes, but not astrocytes, contained mature Slit2. An additional antibody raised against a phylogenetically conserved epitope ofDrosophilaSlit confirmed this finding (Slit). (d–f) Slit2-like immunoreactivity localized to oligodendrocyte somas (s) and processes. Membranous staining pattern is shown in botheandf(arrowheads). Asterisks (*) indicate location of the nucleus. (g,h) Oligodendrocyte differentiation and increased Slit2 immunoreactivity, particularly in end feet (arrowheads), upon JZL184 exposure. (i) Slit2 protein content in oligodendrocytes after JZL184 treatment. (j) JZL184-induced Slit2 accumulation in oligodendrocyte end feet as measured by quantitative morphometry. (k–n) Effect of AM630, a CB2R antagonist, on JZL184-induced Slit2 accumulation in oligodendrocyte end feet (open and closed arrowheads). (o,p) The effect of siRNA-mediated MGL inhibition on Slit2 expression in end feet (arrowheads). (q) CNPase+oligodendroglial end feet in the interbundle space (ibs) and in apposition to enlarged fascicles of Robo1+corticofugal axons (cfa) in JZL184-treated mouse embryos. (r) Three-dimensional reconstruction of Slit2 in oligodendrocyte end feet (arrowheads) adjacent to corticofugal axons. (s) Schematic of JZL184-induced remodelling of axonal pathfinding upon premature oligodendrocyte differentiation. Data were expressed as means±s.e.m.,n=8–32 cells per group for each condition in duplicate experiments; *P<0.05 (Student’st-test). Scale bar, 10 μm (a,h,o,q), 2 μm (m). Figure 6: JZL184 alters Slit2 expression and localization in oligodendrocytes. ( a ) Oligodendrocytes (solid arrowheads), but not astrocytes, (open arrowheads) contained Slit2. ( b ) GFAP and CNPase were used to validate the purity of isolated astrocytes and oligodendrocytes, respectively. ( c ) Oligodendrocytes, but not astrocytes, contained mature Slit2. An additional antibody raised against a phylogenetically conserved epitope of Drosophila Slit confirmed this finding ( Slit ). ( d – f ) Slit2-like immunoreactivity localized to oligodendrocyte somas ( s ) and processes. Membranous staining pattern is shown in both e and f (arrowheads). Asterisks (*) indicate location of the nucleus. ( g , h ) Oligodendrocyte differentiation and increased Slit2 immunoreactivity, particularly in end feet (arrowheads), upon JZL184 exposure. ( i ) Slit2 protein content in oligodendrocytes after JZL184 treatment. ( j ) JZL184-induced Slit2 accumulation in oligodendrocyte end feet as measured by quantitative morphometry. ( k – n ) Effect of AM630, a CB 2 R antagonist, on JZL184-induced Slit2 accumulation in oligodendrocyte end feet (open and closed arrowheads). ( o , p ) The effect of siRNA-mediated MGL inhibition on Slit2 expression in end feet (arrowheads). ( q ) CNPase + oligodendroglial end feet in the interbundle space (ibs) and in apposition to enlarged fascicles of Robo1 + corticofugal axons (cfa) in JZL184-treated mouse embryos. ( r ) Three-dimensional reconstruction of Slit2 in oligodendrocyte end feet (arrowheads) adjacent to corticofugal axons. ( s ) Schematic of JZL184-induced remodelling of axonal pathfinding upon premature oligodendrocyte differentiation. Data were expressed as means±s.e.m., n =8–32 cells per group for each condition in duplicate experiments; * P <0.05 (Student’s t -test). Scale bar, 10 μm ( a , h , o , q ), 2 μm ( m ). Full size image Excess 2-AG facilitates oligodendrocyte differentiation in culture [21] and in vivo ( Fig. 3 ). Here, we show that JZL184 increased Slit2 expression in cultured oligodendrocytes ( Fig. 6g–i ), and increased Slit2-like immunoreactivity in their end feet ( Fig. 6j ). JZL184’s effect on Slit2-like labelling in oligodendroglia end feet was reversed by AM630, a CB 2 R antagonist [21] ( Fig. 6k–n ), suggesting that Slit2 production and subcellular translocation might be regulated by agonist (for example, 2-AG) signalling at CB 2 Rs. To verify the effects of JZL184 on Slit2 production, we transfected cultured oligodendrocytes with MGL siRNA, which recapitulated the increase of Slit2-like immunoreactivity in oligodendrocyte end feet ( Fig. 6o,p ). In JZL184-treated brains, CNPase + /CB 1 R − oligodendroglial end feet juxtaposed Robo1/CB 1 R double-labelled corticofugal axons ( Fig. 6q ), and accommodated enlarged fascicles by forming proportionately larger glial scaffolds (that is, no CNPase labelling within individual fascicles; Fig. 6q ). These oligodendroglia end feet harboured Slit2-like immunoreactivity, which frequently juxtaposed nearby axons ( Fig. 6r ). These data together with Robo1/CB 1 R ( Fig. 5a ) and Robo2/CB 1 R ( Fig. 5a ) co-localization and Robo1/Robo2 mRNA ( Fig. 5b ) and protein ( Fig. 5c ) expression in cultured cortical neurons suggest that endocannabinoids are poised to modulate Slit/Robo signalling, and support a model in which ectopic Slit2 presentation by cortical oligodendrocytes participates in inducing growth errors of CB 1 R + axons in vivo ( Fig. 6s ). JZL184 fails to affect axonal growth in Robo1 −/− mice If focal Robo1/Slit2 interactions are indeed modulated by 2-AG signalling, then JZL184 administration to Robo1 −/− (ref. 42 ) mice will reveal incomplete cortical phenotypes due to the neuron versus oligodendroglia-driven arch of the proposed signalling axis ( Fig. 7a ). Robo1 −/− mice per se present an axon fasciculation phenotype [5] . If Robo1 receptors are downstream from CB 1 Rs, then JZL184 likely would fail to affect the pre-existing axonal phenotype in Robo1 −/− mice. Indeed, the spread of callosal axons [5] ( Fig. 7b ) remained unaffected in JZL184-treated Robo1 −/− mice. As such, neither the diameter of individual and enlarged axon fascicles nor their interbundle distance were affected by JZL184 ( Fig. 7c,d,f ). In contrast, JZL184 provoked CNPase + oligodendroglial end-feet differentiation in Robo1 −/− mice. Yet oligodendroglial end feet were interspersed with individual corticofugal axons, confirming the loss of a chemorepulsive cue ( Fig. 7e,g ). These data dissociate between the loss of CB 1 R-driven and Robo1 receptor-dependent axon guidance deficits and CB 2 R-mediated focal chemorepulsion and oligodendroglial differentiation in vivo . 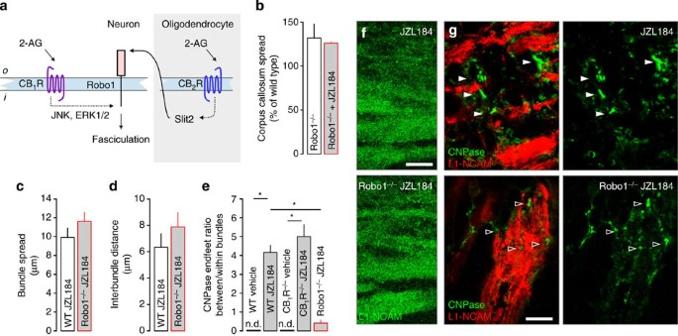Figure 7: JZL184-induced oligodendroglial repositioning in Robo1−/−mice. (a) Schematic overview of 2-AG signalling converging on axonal growth and fasciculation through Slit/Robo signalling. (b) Callosal axon fasciculation in Robo1−/−mice treated with JZL184. Note that untreated Robo1−/−mice presented a fasciculation phenotype5. (c,d) Diameter of individual bundles and their interbundle distance upon JZL184 treatment in Robo1−/−embryos. (e–g) Oligodendroglia end-feet infiltrated axonal bundles in JZL184-treated Robo1−/−mice. This was undetected (ND) in wild-type or CB1R−/−embryos. Data were expressed as means±s.e.m., fromn=3–5 embryos per genotype; *P<0.05 versus respective wild-type (WT) controls (Student’st-test). Scale bar, 10 μm (f,g). Figure 7: JZL184-induced oligodendroglial repositioning in Robo1 −/− mice. ( a ) Schematic overview of 2-AG signalling converging on axonal growth and fasciculation through Slit/Robo signalling. ( b ) Callosal axon fasciculation in Robo1 −/− mice treated with JZL184. Note that untreated Robo1 −/− mice presented a fasciculation phenotype [5] . ( c , d ) Diameter of individual bundles and their interbundle distance upon JZL184 treatment in Robo1 −/− embryos. ( e – g ) Oligodendroglia end-feet infiltrated axonal bundles in JZL184-treated Robo1 −/− mice. This was undetected (ND) in wild-type or CB 1 R −/− embryos. Data were expressed as means±s.e.m., from n =3–5 embryos per genotype; * P <0.05 versus respective wild-type (WT) controls (Student’s t -test). Scale bar, 10 μm ( f , g ). Full size image Slit2/Robo1 signals mediate JZL184-induced chemorepulsion We devised a genetically amenable co-culture system to show that Slit2 + oligodendrocytes affect directional growth decisions of Robo1 + /CB 1 R + neurites in vitro . Neurites regularly contacted oligodendrocytes under control conditions ( Fig. 8a ). JZL184 administration in vitro enhanced Slit2 expression and mobilized Slit2 to submembranous positions in oligodendrocytes ( Fig. 8b ), with coincident repulsive responses of nearby neurites as shown by their increased distance to apposing glial surfaces (15.65±1.01 μm (JZL184) versus 9.74±1.11 μm (vehicle), P <0.05; Fig. 8d ). 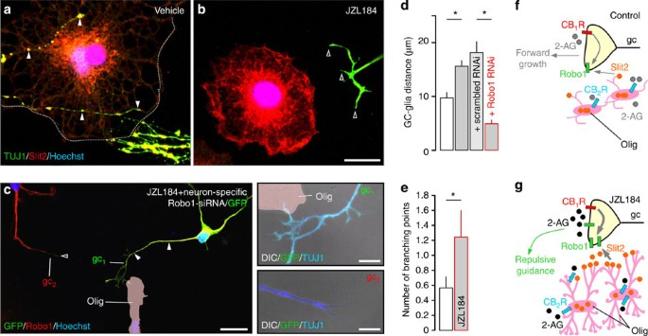Figure 8: JZL184 induces growth cone repulsion via Slit2/Robo1 signalling. (a) Neurites (arrowheads) contacting oligodendrocytes when co-cultured. (b) Neurites (open arrowheads) excluded from the vicinity of oligodendrocytes upon JZL184 application. Note the intensely Slit2+peripheral domain of the oligodendrocyte (Olig) shown. (c) A neurite (arrowheads) of a Robo1 siRNA/GFP co-transfected neuron (gc1in green), but not of a non-transfected neuron (gc2in red), overcame chemorepulsion. Insets (gc1,gc2) depict high-resolution images of the growth cones shown in (c). (d) Growth cone distances to the most proximal surface of the nearest oligodendrocyte. (e) JZL184 induced branching of neuronal processes in the vicinity of oligodendrocytesin vitro. (f,g) Schema of Slit2/Robo1 signalling downstream from cannabinoid receptors. Data were expressed as means±s.e.m., triplicate experiments withn=3 samples run in parallel;n=6–9 observations per group. *P<0.05 (Student’st-test). Scale bar, 8 μm (a1,b), 3 μm (insets). Figure 8: JZL184 induces growth cone repulsion via Slit2/Robo1 signalling. ( a ) Neurites (arrowheads) contacting oligodendrocytes when co-cultured. ( b ) Neurites (open arrowheads) excluded from the vicinity of oligodendrocytes upon JZL184 application. Note the intensely Slit2 + peripheral domain of the oligodendrocyte (Olig) shown. ( c ) A neurite (arrowheads) of a Robo1 siRNA/GFP co-transfected neuron (gc 1 in green), but not of a non-transfected neuron (gc 2 in red), overcame chemorepulsion. Insets (gc 1 ,gc 2 ) depict high-resolution images of the growth cones shown in ( c ). ( d ) Growth cone distances to the most proximal surface of the nearest oligodendrocyte. ( e ) JZL184 induced branching of neuronal processes in the vicinity of oligodendrocytes in vitro . ( f , g ) Schema of Slit2/Robo1 signalling downstream from cannabinoid receptors. Data were expressed as means±s.e.m., triplicate experiments with n =3 samples run in parallel; n =6–9 observations per group. * P <0.05 (Student’s t -test). Scale bar, 8 μm (a 1 ,b), 3 μm (insets). Full size image We used siRNA knockdown of Robo1 in neurons co-cultured with oligodendrocytes in the presence of JZL184 for 4 days to test whether JZL184-mediated neurite repulsion relied on Robo1 receptors. Co-transfection with a GFP plasmid and post hoc labelling for Robo1 receptors ( Supplementary Fig. 5c ) confirmed successful neuronal Robo1 silencing. Robo1 knockdown overcame JZL184-induced repulsion and adopted differentiated growth cone morphologies ( Fig. 8c ). Consequently, neurites of Robo1 siRNA-transfected neurons approached oligodendrocytes, leaving the growth cone-oligodendrocyte distance significantly reduced (4.97±0.69 μm (Robo1 siRNA) versus 18.21±2.06 μm (scrambled siRNA), P <0.05; Fig. 8d ). Further, JZL184 administration increased the number of branching points on approaching neurites in the close vicinity of oligodendocytes ( Fig. 8e ), suggesting that an increased number of axon collaterals might, at least in part, contribute to changes in callosal microanatomy. Cumulatively, these data identify endocannabinoids as candidates to upstream regulate Slit2/Robo1 interactions during directional axonal growth ( Fig. 8f,g ). Endocannabinoids affect neuronal differentiation, including directional axonal growth during corticogenesis [17] , [19] , [43] . Endocannabinoid signalling appears particularly efficacious to modulate axonal growth since CB 1 Rs are selectively enriched in navigating axons, and are co-targeted with DAGLs to advancing growth cones [30] , [43] . Establishment of major axonal tracts critically relies on chemorepulsive Slit gradients [4] , [5] , [7] . In fact, midline crossing of commissural axons particularly depends on focal Slit/Robo signalling between neurons and glia [44] . The architecture of corticofugal axons is altered in CB 1 R −/− mice [18] , a phenotype reminiscent to those of Robo1 −/− /Robo2 −/− mutants [4] . Here, we resolve this similarity by dissecting a molecular interplay between endocannabinoids and the Slit/Robo signalling axis. Our data suggest that the lack of CB 1 R-induced Robo1 accumulation in growth cones might disrupt, at least in part, axonal navigation and contribute to the altered topography of corticofugal axons in CB 1 R −/− mice. However, by showing that increased 2-AG levels upon MGL inhibition coincidently induce CB 2 R-mediated oligodendrocyte differentiation and CB 1 R-dependent axonal misrouting in the corpus callosum, we characterize an intercellular signalling network in which a single endocannabinoid ligand engages molecularly distinct cannabinoid receptors in neurons and glia to upstream control chemorepellent production (Slit2 in glia) and signalling (Robo1 in neurons). Whether changes in axonal topography in the corpus callosum of JZL184-treated mice reflect an increased number of axon collaterals or instead are due to the spatial reorganization of the same number of axons (because of, for example, changes to extracellular matrix composition) as in controls remains unknown. Our in vitro data on the JZL184-induced increase of neurite branching points supports the former scenario, and suggests that an increased numbers of axon collaterals compacting in callosal fascicles might significantly increase network instability due to erroneous synaptic wiring. Our results in cultured neurons are also compatible with those from Robo1 −/− mutant embryos, where glial repositioning around enlarged axon fascicles could argue for the disruption of a critical glial–neuronal signal interface. We employed JZL184, a selective MGL inhibitor [23] , to increase endocannabinoid levels in the fetal brain. The selectivity of this compound was verified using activity-based protein profiling after in vivo drug application, as well as in in vitro experiments using genetically or RNA-silenced primary cultures. Since JZL184 application does not desensitize CB 1 R unless used for extended periods [36] , our data suggest that ectopic, cell type- and cannabinoid receptor subtype-dependent signalling events took place in JZL184-exposed fetuses, sufficient to affect axonal growth and guidance. This included an increased transport of Robo1 along the axon culminating in peak expression levels and externalization in the growth cone, likely modulated via mitogen-activated protein kinase and JNK signalling, as well as an increased Slit2 expression on an enlarged oligodendroglial end-feet arbour. Considering that CB 1 Rs are broadly distributed in the developing nervous system [45] , [46] , including descending projections to the spinal cord [45] , [47] , our results might have profound implications for the overall organization of axonal connectivity in the nervous system. Although we did not seek to identify the cellular origin of signal-competent 2-AG, a number of alternative sources may exist. These include the elongating corticofugal axons themselves, which contain DAGLα (and β) [17] , [18] . If so, Slit2/Robo1 signalling might represent a cell-autonomous amplification mechanism whereby DAGL-derived 2-AG could activate CB 1 Rs within growth cones [30] , facilitating Robo1 trafficking. Recent data suggest that 2-AG can diffuse extracellularly and evoke physiological responses in a radius of 20–100 μm (refs 48 , 49 ). Thus, DAGL activity in axonal growth cones appears sufficient to generate focal 2-AG microgradients to activate CB 2 Rs on neighbouring oligodendrocytes to stimulate Slit2 production and release ( Fig. 8f,g ). At the level of signal transduction, CB 1 Rs and Robo1/2 can coordinately activate downstream effectors within axonal growth cones, which can act as reinforcers of the individual receptors’ signal outputs. Members of the Rho family of GTPases, which can be activated by either receptor in various tissues [19] , [50] , [51] and whose activity is indispensable for cytoskeletal instability allowing growth cone motility [52] , can be central to orchestrating endocannabinoid-induced modifications to cytoskeletal remodelling during repulsive growth cone turning. An advantage of this model, combining elements of autocrine endocannabinoid and paracrine Slit2/Robo1 signalling, is that it ascertains the ‘on-demand’ upstream coupling of endocannabinoids to Slit2/Robo1 signalling, outlining a temporally defined, spatially restricted and highly dynamic mechanism to modulate growth cone-steering decisions. We also show that CB 1 R–Robo1 receptor co-localization is preserved during mammalian evolution, as evidenced by our histochemical data from midgestational human fetuses. Moreover, Robo1 and Slit mRNA expression in human fetal brains are developmentally regulated and appear tightly coupled. Maternal cannabis smoking significantly increased the amount of Robo1 mRNA in the human fetal cerebrum. We propose that the molecular re-configuration of Slit/Robo signalling networks by phytocannabinoids via the CB 1 R can be a candidate molecular mechanism to explain altered synaptic neurotransmission, and consequently, behavioural and cognitive deficits in children exposed in utero to cannabis [53] , [54] . Considering the continued increase of cannabis smoking during adolescence [41] , the erroneous recruitment of spatially segregated CB 1 Rs and CB 2 Rs to regulate Slit2/Robo1 interactions during the postnatal refinement of neuronal circuits might also introduce unwanted modifications to the cortical wiring diagram. Besides cannabis, fetal infections are associated with the induction of endocannabinoid signalling in placental macrophages, contributing excess endocannabinoids to the fetal circulation [55] . This cascade can change the temporal and subcellular recruitment of CB 1 Rs and CB 2 Rs, imposing pathological challenges on the signalling mechanism we uncovered. Overall, we suggest that a hierarchical interplay between endocannabinoid and Slit/Robo signalling networks is a primary regulatory node in the developing corticofugal system. Animals and tissue preparation Tau gfp/gfp ::CB 1 R −/− mice were generated by first crossing tau gfp/+ and CB 1 R −/+ mice (both on C57BL/6 background) to select tau gfp/+ ::CB 1 R −/+ colony founders. Next, we crossed heterozygous offspring to generate tau gfp/gfp ::CB 1 R −/+ parents for in vivo analysis. Given that tau is dispensable for neuronal development, tau gfp/gfp mice did not carry any developmental abnormality [29] . We used mice heterozygous for CB 1 Rs as parents throughout the experiments, allowing direct comparison of littermate tau gfp/gfp ::CB 1 R −/− and tau gfp/gfp ::CB 1 R +/+ offspring. MGL +/+ and MGL −/− littermates of both sexes from heterozygous pregnancies [23] were analysed on E16 and postnatal day (P)20 ( Supplementary Fig. 1 ). Pregnant CB 1 R −/+ , tau gfp/gfp ::CB 1 R −/+ , Robo1 −/+ [5] , Slit2 +/− [56] and wild-type C57BL/6 mice were injected with JZL184 (40 mg kg −1 body weight, intraperitoneally daily) [24] or vehicle intraperitoneally during E12.5–18.5. Male mouse embryos ( n >6/pregnancy, n >2 pregnancies/analysis) were collected at E18.5. Whole brains were collected for histochemistry, protein biochemistry/western blotting, mass spectrometry, JZL184-binding assay or quantitative RNA profiling. Experiments on live animals conformed to the 86/609/EEC directive and were approved by the regional authority (Stockholm Norra Djuretiska Nämnd; N512/12). Human fetal tissue preparation and histochemistry Three fetal brains with normal development (between 20–23 gestational weeks) were selected from the Brain Bank of the Institute of Neurology, Medical University of Vienna, Austria. Fetal brain tissue was obtained from spontaneous or medically induced abortions. Only cases without genetic disorders, head injury or neurological diseases were included. These cases showed no chromosome aberrations or post-mortem autolysis. Neuropathological examination excluded major central nervous system malformations, severe hypoxic/ischaemic encephalopathy, intraventricular haemorrhages, severe hydrocephalus and meningitis or ventriculitis. Demographic data are summarized in Supplementary Table 3 . Tissues were obtained and used compliant with the Declaration of Helsinki and following institutional guidelines. The study was performed in the course of an approved study by the Ethical Committee of the Medical University of Vienna (No.104/2009). Immunohistochemistry, imaging and quantitative morphometry Embryonic brains were immersion fixed in 4% paraformaldehyde in phosphate buffer (0.1 M, pH 7.4, PB) overnight. Tissue samples were cryoprotected in 30% sucrose in physiological saline for at least 48 h before cryostat serial sectioning (16 μm thickness), and thaw-mounted on SuperFrost + glass slides. Multiple immunofluorescence histochemistry was carried out according to published protocols [19] , [57] . Sections were washed in PB and pre-treated with 0.3% Triton X-100 (in PB) for 1 h at 22–24 °C to enhance the penetration of primary antibodies. Non-specific immunoreactivity was suppressed by incubating our specimens in a cocktail of 10% normal donkey serum (Jackson), 5% bovine serum albumin (Sigma) and 0.3% Triton X-100 (Sigma) in PB for 1 h at 22–24 °C. Sections were exposed (16–72 h at 4 °C) to select combinations of primary antibodies ( Supplementary Table 1 ) diluted in PB to which 0.1% normal donkey serum and 0.3% Triton X-100 had been added. After extensive rinsing in PB, immunoreactivities were revealed by carbocyanine (Cy)2, 3 or 5-tagged secondary antibodies raised in donkey (1:300 (Jackson), 2 h at 22–24 °C). Hoechst 33342 (Sigma), a nuclear dye, was applied to reveal tissue architecture. Sections were coverslipped with Dako Fluorescent mounting medium (Dako). Sections were inspected and images acquired on a 710LSM confocal laser-scanning microscope (Zeiss). Image surveys were generated using the tile scan function at × 10 primary magnification (Plan-Neofluar × 10/0.30). High-resolution images were acquired with optical zoom ranging from × 1.5–3.0 at × 63 primary magnification (Plan-Apochromat × 63/1.40, and 0.5–0.7 μm optical slice thickness) to limit signal detection. Emission spectra for each dye were limited as follows: Cy2 (505–530 nm), Cy3 (560–610 nm) and Cy5 (650–720 nm). The coexistence of immunosignals was verified by capturing serial orthogonal z -image stacks at × 63 primary magnification (up to × 3 optical zoom) and accepted if these were present without physical signal separation in ≤1.0-μm optical slices, and overlapped in all three ( x , y and z ) dimensions within individual cellular domains. Morphometric analysis of fetal mouse brains was aided by the ZEN2010 software and included: (i) the transverse diameter (μm) of L1-NCAM + corticofugal axons (‘corpus callosum spread’) in fetal wild-type and CB 1 R −/− and MGL −/− brains after JZL184 or vehicle administration, (ii) the density and (iii) proximity (μm) of first-order fascicles of >3 μm in diameter, (iv) the density ( n ), (v) diameter (μm), (vi) embedding of CNPase + oligodendrocyte end-feet interspersing callosal axons and (vi) calibrated fluorescence intensities using an arbitrary grey-scaled unit scale in images acquired with identical laser illumination and capture settings. Robo1 receptor immunoreactivity along growth cones and axons of primary cortical neurons was measured in ImageJ 1.45 s (NIH). Validation of the Slit2 antibody was performed on 600-nm-thin serial optical slices of embryonic brain sections obtained from Slit2 −/− and littermate wild-type mice. The number of Slit2 + profiles was counted and their density calculated on CNPase + oligodendrocyte end feet or perinuclear loci. Multi-panel images were assembled in CorelDraw X5. Human fetal immunohistochemistry and analysis Three-micrometer tissue sections of formalin-fixed, paraffin-embedded tissue blocks containing the corpus callosum and the hippocampal formation were mounted on pre-coated glass slides (Star Frost) [58] , [59] . Shortly, after deparaffinization and rehydration, the sections were pre-treated in low pH EnVision FLEX antigen retrieval solution at 98 °C for 20 min (PTLink; Dako) and subsequently incubated with rabbit anti-Robo1 (ab7279; Abcam; 1:500) or guinea pig anti-CB 1 R (Dr M. Watanabe 1:1,000) antibodies. The DAKO EnVision detection kit, peroxidase/DAB and rabbit/mouse (K5007, ready-to-use, Dako) was used to visualize antibody binding. Sections were counterstained with haematoxylin, dehydrated in ascending concentrations of ethanol, cleared with xylene and covered with Consil-Mount (Shandon; Thermo Scientific). Representative images containing the area of interest were exported from scanned sections (NanoZoomer 2.0, Hamamatsu). For immunofluorescent co-localizations, 5-μm-thick sections were pre-treated with 1% sodium borohydride, rinsed extensively in 25 mM Tris-Buffer (pH 7.5) and blocked in 20% normal horse serum (Vector Laboratories) for 30 min. Mixtures of primary antibodies were applied for 48 h at 4 °C (anti-Robo1 diluted 1:500 and anti-CB 1 R diluted 1:1,000). A mix of secondary antibodies conjugated with Alexa Fluor 488 (Invitrogen/Molecular Probes; 1:1,000) and DyLight 650 (Jackson; 1:400) was applied for 2 h at room temperature. The antibodies were tested for optimal dilution, and secondary antibodies were tested for cross-reactivity and non-specific staining. Sections were imaged and analysed using a Zeiss LSM780 confocal microscope. Western blotting Tissue samples were lysed in modified radioimmunoprecipitation assay buffer containing 1 mM NaF, 1 mM Na 3 VO 4 , 0.1% N -octyl-β- D -glucopyranoside and a mixture of protease inhibitors (Complete, Roche). Cell debris and nuclei were pelleted by centrifugation (800 g , 10 min at 4 °C). Protein concentrations were determined by Bradford’s colorimetric method [60] . Samples were diluted to a final protein concentration of 2 μg μl −1 , denatured in 5 × Laemmli buffer and analysed by SDS–polyacrylamide gel electrophoresis on 6 or 8% resolving gels. After transferring onto Immobilon-FL polyvinylidene difluoride membranes (Millipore), membrane-bound protein samples were blocked in 3% bovine serum albumin and 0.5% Tween-20 diluted in Tris-buffered saline for 1.5 h, and subsequently exposed to primary antibodies ( Supplementary Table 1 ; Supplementary Fig. 7 ) overnight at 4 °C. Appropriate combinations of horseradish peroxidase-conjugated secondary antibodies (Jackson; from goat, rabbit, guinea pig or mouse hosts; 1:10,000 for 2 h) were used for enhanced chemiluminescence signal detection. Image acquisition and analysis were performed on a Bio-Rad XRS + imaging platform. TUJ1 served as loading control, which showed corresponding quantities of β-actin and gapdh ( Supplementary Fig. 4f ). PCR To discriminate the sex of mouse fetuses, we used primers to amplify Y and X chromosome-specific genomic DNA sequences. The Sry gene (forward: 5′-GTTCAGCCCTACAGCCACAT-3′, reverse: 5′-CAGCTGCTTGCTGATCTCTG-3′, amplicon size: 197 bp (Y chromosome)) and DXNds3 microsatellite (forward: 5′-GAGTGCCTCATCTATACTTACAG-3′, reverse: 5′-TCTAGTTCATTGTTGATTAGTTGC-3′, amplicon size: 244 bp (X chromosome)) were amplified. For quantitative PCR, E18 embryonic mouse brains were microdissected on ice to isolate pallial regions, and snap frozen in liquid N 2 until processing. RNA was extracted using the RNeasy mini kit (Qiagen) with a DNase I step performed to eliminate traces of genomic DNA [30] and reverse transcribed using a high-capacity cDNA reverse transcription kit (Applied Biosystems). Reactions were performed after an initial denaturation at 95 °C for 10 min followed by 40 cycles of 95 °C for 15 s denaturation, annealing and extension at calculated temperatures (60 s) and a dissociation stage (from 60 to 95 °C with 0.5-°C steps for 10 s each; MyiQ Apparatus, Bio-Rad), with primer pairs amplifying short fragments for each gene ( Supplementary Table 2 ). Samples without template or reverse transcriptase served as negative controls. Expression levels were normalized to the housekeeping gene (HKG) encoding glyceraldehyde-3-phosphate dehydrogenase ( gapdh ) obtained for every sample in parallel assays [15] . Human fetal NanoString analysis Midgestational fetal brain subjects (18–22 weeks of gestation), collected after saline-induced elective abortions under Institutional Review Board approval at SUNY Downstate Medical Center, Brooklyn, New York, were fixed in 1% paraformaldehyde in 0.05 M PB for 24 h, frozen in dry ice-cooled isopentane, cryosectioned in the coronal plane (20 μm) and stored at −30 °C (ref. 61 ). Tissue isolations from the cortex were carried out with micro-RNAqueous lysis solution (Life Technologies) and gene expression analysed using the nCounter System from NanoString Technologies [62] at the Gene Expression Shared Resource Facility at Icahn School of Medicine. Briefly, the cell lysates were hybridized to a NanoString code-set containing barcode-labelled probes for ROBO1, SLIT1 and three HKGs: TBP , Hsp90ab1 and ActB ( Supplementary Table 4 ), followed by scanning of the immobilized mRNA transcripts in the nCounter Digital Analyzer. The raw data files were normalized to the TBP HKG via NanoString nCounter software, and statistical analysis was performed using the JMP statistical program (SAS Institute, Cary, NC). A general linear stepwise regression was used to calculate statistical significance and identify covariates. Variables were clustered as (i) fetal age, (ii) fetal body weight and foot length (‘developmental measures’) and (iii) cannabis exposure. A univariate model was first performed with each cluster of variables and any variable that showed P <0.10 was included in the stepwise regression, in addition to cannabis exposure addition [61] . Variables with P <0.05 were included in the final regression model as covariates of cannabis exposure. Liquid chromatography tandem mass spectrometry 2-AG, anandamide (AEA), 2-linoleoyl glycerol and oleoylethanolamide concentrations were determined using a solid-phase extraction liquid chromatography tandem mass spectrometry method [30] , [63] . The final JZL184 (40 mg kg) injection was given to pregnant females on E18.5 2 h before dissection of maternal and fetal brains. Embryonic hemisected brains ( n =6 pups from two separate litters) were homogenized in ice-cold acetonitrile containing [ 2 H 4 ]anandamide at 6 pmol as internal standard, made up to 70% water and centrifuged at 13,000 r.p.m. for 5 min. The supernatant was applied to Strata-X polymeric reverse-phase cartridges (Phenomenex), methanol-eluted analytes were dried under N 2 and the residue was re-suspended in the mobile phase. A Surveyor LC system coupled to a TSQ Quantum mass spectrometer (Fisher Thermo Scientific) was used for analysis. The analytes were eluted from an ACE 5-μ C8 column (150 × 2.1 mm; Hichrom Ltd.) under isocratic conditions with a mobile phase consisting of 15% water, 85% methanol and 0.5% formic acid at a flow rate of 200 μl min −1 at 30 °C. Mass spectrometry analysis was performed using electrospray ionization in positive ion mode. Quantification was undertaken using single-reaction monitoring of the parent ion–product ion transitions for 2-AG and [ 2 H 4 ]AEA of mass-to-charge ratio ( m / z ) of m / z 379 to m / z 287 and m / z 352.2 to m / z 66.2, respectively. Two peaks were present in the chromatogram for 2-AG because a 1(3)-isomer exists in equilibrium with 2-AG. The areas of both peaks were combined to calculate [2-AG] by weighted linear regression analysis against suitable calibration standards using Xcalibur 2.0.6 software (Fisher Thermo Scientific). Results were expressed as nanomoles/picomoles per gram of tissue. Ex vivo activity-based protein profiling Frozen, hemisected brains from E18.5 mouse embryos (~35 mg; other hemisphere from mass spectrometry analysis) or a section of the cortex from the corresponding mother (~90 mg) were washed with cold Dulbecco’s phosphate-buffered saline (DPBS) (2 × 1.0 ml) and homogenized using a Branson Sonifier 250 probe sonicator (10 pulses, 50% duty cycle, output setting=3.0) in cold DPBS (10 μl mg −1 tissue). Homogenates derived from adult mouse brain samples were centrifuged (3,000 g , 3 min) at 4 °C and the pellet was discarded. The total protein concentration for each tissue homogenate was then determined using the DC Protein Assay (Bio-Rad), and each proteome was diluted to 1.0 mg ml −1 in DPBS. Proteomes (50 μl) were subsequently treated with FP-Rhodamine (1.0 μl, 50 μM in DMSO), incubated for 30 min at room temperature and quenched with 4 × SDS loading buffer (17 μl). Following separation of proteins by SDS–polyacrylamide gel electrophoresis (10% acrylamide gel) and fluorescent gel imaging (Hitachi FMBio II flatbed scanner), serine hydrolase activities were determined by measuring the fluorescent intensity of target gel bands using ImageJ 1.45s (ref. 24 ). Primary cultures, pharmacology and transfection The pallium of embryonic mice was dissected at E16.5. For neuronal cultures, cortical cells from C57BL/6 and CB 1 R −/− mice were enzymatically dissociated and plated at a density of 25–50 000 cells per well (morphometry) or 10 6 cells per ell (biochemistry) in poly- D -lysine-coated 24-well or 6-well plates, respectively [30] . Primary neuron cultures were maintained in Dulbecco’s modified Eagle’s medium (DMEM)/F12 (1:1) containing B27 supplement (2%), L -glutamine (2 mM), penicillin (100 U ml −1 ) and streptomycin (100 μg ml −1 ; all from Invitrogen) and exposed to drugs applied alone or in combination (JZL 184: 100 nM, Cayman Chemical; O-2050: 200 nM, Tocris Bioscience; AM630: 200 nM, Tocris Bioscience; AM251: 200 nM, Tocris Bioscience; UO126: 10 μM, Tocris Bioscience; SP600125: 5 μM, Tocris Bioscience). Primary cortical neurons from C57BL6/N fetuses were transfected on 1 day in vitro by Lipofectamine 2000 (5 μl; Invitrogen) with a pool of MGL-specific siRNAs (sc-72278; 50 pmol per well) or non-targeting siRNA (sc-36869; 50 pm per well; Santa Cruz Biotechnology) for 30 min. Neurons were left to recover for 3 days before fixation in 4% paraformaldehyde. For glial cultures, neocortices of P2 mouse pups were dissected. Cells were dissociated similarly, transferred to T75 flasks (3 × 10 7 cells per flask) and maintained in DMEM containing 10% fetal bovine serum, L -glutamine (2 mM), penicillin (100 U ml −1 ) and streptomycin (100 μg ml −1 ). After 7–9 days, T75 flasks were placed on a shaker at 190 r.p.m. at 37 °C for 1 h. The microglial fraction was discarded and cells were allowed to equilibrate for 2–6 h in fresh medium. Subsequently, flasks were placed onto an orbital shaker at 210 r.p.m., 37 °C for 16–18 h to separate oligodendrocytes. The supernatant (oligodendroglial fraction) was collected, centrifuged, re-suspended and seeded at a density of 25,000 cells per well (morphometry) and 10 6 cells per well (biochemistry) in poly- D -lysine-coated 24-well and 6-well plates, respectively. Cultures were then treated with JZL184 (100 nM) every other day for 72 h or with MGL-specific siRNA/non-targeting siRNA as described above. Cell pellets from the same fraction were taken and processed for western blotting and PCR analysis simultaneously. Astrocytes were collected in fresh medium and processed for protein and mRNA analyses. For neuron–glia co-cultures, oligodendrocytes were plated at a density of 25,000 cells per well in DMEM containing 10% fetal bovine serum. After 1 day, half of the medium was removed and replaced by DMEM/F12 (1:1) culture medium supplemented with B27 (2%) and neurons were seeded at a density of 25,000 cells per well. In another set of experiments, Lipofectamine 2000 (5 μl; Invitrogen) was used to transfect co-cultures with either non-targeting (scrambled) siRNA (sc-36869) or a pool of Robo1-specific mouse siRNAs (sc-42253; both at 100 pmol per well; Santa Cruz Biotechnology) for 4 h. Co-cultures were treated with JZL184 (100 nM) every other day for 72 h. Cells on coverslips were immersion fixed on ice with 4% paraformaldehyde in 0.1 M PB and processed as above for immunocytochemistry. Morphological parameters were determined by analysing calibrated images in the ZEN2010 imaging software module (Zeiss; n >30 cells per group) [18] , [30] . In primary neuronal cultures, the intensity of Robo1 and Robo2 imunoreactivities along the neurite ( n >20 per marker and experimental group on two coverslips of two independent experiments each) was measured by obtaining a plot profile starting at the growth cone and continuing along the total axon back to the soma. In primary oligodendrocyte cultures, Slit2 immunoreactivity was measured in end feet and along processes ( n >30 cells per group on two coverslips from duplicate experiments). Immunoreactivity was normalized to vehicle-treated end feet. Distances between neurites and oligodendrocytes were measured in neuron–glia co-cultures ( n >20/ group on two coverslips from duplicates). GCP isolation Cortical hemispheres from E18.5 mouse embryos ( n =5 embryos per treatment) were vibratome sectioned (200–300 μm thickness), pooled ( n =5 embryos per treatment) and exposed to JZL184 (100 nM in DMEM/F12/B27 as above) for 25 or 80 min at 37 °C in vitro . Control samples were incubated with vehicle for 80 min. GCPs were isolated from vehicle- or JZL184-treated samples according to published protocols [64] . Robo1 protein levels of GCPs were determined by western blotting ( Supplementary Table 1 ). β-III-tubulin served as internal loading control [30] . Statistics Data were analysed using Statistical Package for the Social Sciences (version 21.0, SPSS Inc.). Pair-wise group comparisons in histochemical and western blotting experiments were evaluated using the Student’s t -test (on independent samples). Data were normalized to controls as indicated. Data were expressed as means±s.e.m. A P -value of 0.05 was considered statistically significant. How to cite this article: Alpár, A. et al . Endocannabinoids modulate cortical development by configuring Slit2/Robo1 signalling. Nat. Commun. 5:4421 doi: 10.1038/ncomms5421 (2014).